Switching plastic crystals of colloidal rods with electric fields When a crystal melts into a liquid both long-ranged positional and orientational order are lost, and long-time translational and rotational self-diffusion appear. Sometimes, these properties do not change at once, but in stages, allowing states of matter such as liquid crystals or plastic crystals with unique combinations of properties. Plastic crystals/glasses are characterized by long-ranged positional order/frozen-in-disorder but short-ranged orientational order, which is dynamic. Here we show by quantitative three-dimensional studies that charged rod-like colloidal particles form three-dimensional plastic crystals and glasses if their repulsions extend significantly beyond their length. These plastic phases can be reversibly switched to full crystals by an electric field. These new phases provide insight into the role of rotations in phase behaviour and could be useful for photonic applications. Owing to their size, colloidal particles are an interesting model system for condensed matter, because Brownian motion ensures that the phase behaviour is analogous to that of atomic and molecular systems [1] , [2] and particle coordinates can be obtained quantitatively in three-dimensional (3D) real space on a single particle level [3] , [4] , [5] , [6] . In addition to the system being able to reach equilibrium on experimental time scales, the interaction potentials between the particles can be tuned extensively [6] . For instance, rod-like and plate-like particles have a nematic liquid crystal phase where translational order is short ranged, and there is unconstrained 3D translational motion, but one orientational degree of freedom is still long ranged [1] . This combination of properties makes liquid crystals perfectly suitable for display applications. As such liquid crystals are the positional-rotational opposite of plastic crystals (PCs). The term ‘plastic crystals’ was chosen by Timmermans [7] when he found that some of the molecular plastic crystals could not even support their own weight as a direct consequence of the reduced strength of this solid phase of matter by the rotational dynamics of the molecules on their lattice [7] , [8] . Colloidal liquid crystals are well known [9] ; plastic crystals, however, have hardly been studied experimentally, despite their intriguing structure and dynamics, which are a mixture of those of a liquid and those of a solid. In recent experiments two-dimensional (2D) plastic crystals have been found [10] , [11] , but, as the dimension affects dynamics and structure strongly, these are not the same as 3D systems. For instance, 2D crystals do not have long-ranged order, and a system of disks does not have a glass transition. The only work we are aware of that mentions a 3D colloidal plastic crystal is the recent work by Zukoski et al . [12] They studied slightly anisotropic ‘dicolloids’ for which the shape closely approximated two interpenetrating spheres by x-ray scattering. For certain parameters, it was concluded that a plastic crystal with a long-ranged positional, but random orientational, order had formed. However, because only static scattering experiments were performed, the question of rotations of the particles on their lattice sites on experimental time scales could not be addressed, which leaves open the possibility that the random orientations of the dicolloids were actually frozen in. Such plastic crystals are perhaps better characterized as ‘aperiodic crystals’, as they have sharp diffraction peaks but no true lattice periodicity due to the absence of rotations on an experimental time scale [13] . Similar to the particles as in ref. 12 , almost all molecular plastic crystals for which rotation around one or more axes is possible [7] , [8] consist of an almost spherical shape around their rotation axis (for some examples, see refs 14 , 15 , 16 ). Here we take advantage of the possibility to realize extremely long-ranged repulsions in colloidal systems. By making this range longer than the rods, we demonstrate that even for colloidal rods of 3.3 μm length and a length/diameter ( L / D) ratio as large as 5.6 plastic crystals and, at higher densities, plastic glasses are found in a large range of volume fractions. We also demonstrate by scattering experiments, described later, that field-induced switching of these new plastic crystal phases offers new opportunities for photonic applications. Charged colloidal rods We and others have shown previously for spherical colloids that it is not difficult to achieve electrostatic screening lengths (κ −1 ) of several micrometer in solvents with a relative dielectric constant approximately in between 4 and 10 (refs 6 , 17 ). In this study, we used a recently developed fluorescent model system of micron-sized colloidal silica rods that can be fluorescently labelled [18] and dispersed in the index matching solvent cyclohexylchloride (CHC). In addition to carrying a negative charge (surface potential −70 mV), the colloidal silica rods were sterically stabilized by grafting with short C18 alkane chains and almost index-matched to reduce van der Waals forces and allow for quantitative confocal microscopy measurements >100 μm deep inside the sample. We studied three different rod lengths from 2.3 to 3.3 μm and aspect ratios from 3.8 to 5.6 (see Methods). For relatively high concentrations of an added salt, and thus short screening lengths, nematic and smectic liquid crystal phases were found (not shown here) in accordance with a recent real space study of our group [19] . On the other hand, at low concentrations of salt, the effective repulsive interactions between the rods should become increasingly less anisotropic. On the basis of results of spherical particles [6] , [20] , we expected to obtain crystals with a body centred cubic (BCC) structure in which the rods have the freedom to rotate. The screening lengths for the systems studied in Figs 1 , 2 , 3 , 4 , 5 were maximized by extensively deionizing the solvent to reach screening lengths of about 5 μm, as determined from the conductivity. Apparently, this screening length was sufficient to result in plastic crystals over a range of volume fractions ϕ as is shown by the relatively large region denoted as ‘plastic BCC’ in Figs 1 , 2 , 3a . In the following, we first describe the structures observed without an external electric field. 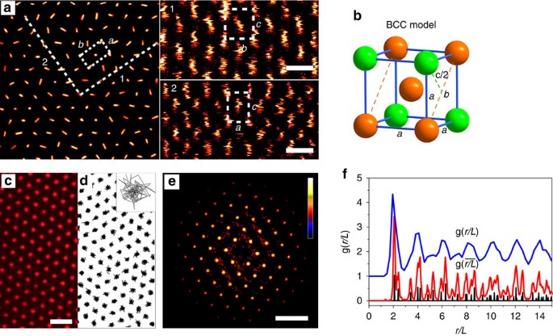Figure 1: Body centred cubic plastic crystal structure. Silica rods R1 withϕ=0.005. (a) Confocal images of a BCC plastic crystal, left: (110) plane; top right: (001) plane; bottom right: (10) plane. The images for the (001) and (10) planes were reconstructed from the same x-y-z stack. (b) Schematic BCC model defining the lattice vectors shown in (a) and (b). (c) The average of 150 frames was measured over a time of 300 s. (d) The corresponding trajectories of particle centres during that time; the inset highlights the trajectory of a single rod. (e) Fourier transform calculated from the monochrome real space image of (c) and (d). The colour bar indicates the logarithmic intensity scale. (f) Pair correlation function g(r) found, from top to bottom, by calculating the g(r) of a single frame, by calculating the g(r) of the average of 150 frames, and from a perfect BCC lattice. The scale bars in (a) and (c) represent 10 μm, and in (e) represents 0.628 μm−1. Figure 1: Body centred cubic plastic crystal structure. Silica rods R1 with ϕ =0.005. ( a ) Confocal images of a BCC plastic crystal, left: (110) plane; top right: (001) plane; bottom right: (10) plane. The images for the (001) and (10) planes were reconstructed from the same x-y-z stack. ( b ) Schematic BCC model defining the lattice vectors shown in ( a ) and ( b ). ( c ) The average of 150 frames was measured over a time of 300 s. ( d ) The corresponding trajectories of particle centres during that time; the inset highlights the trajectory of a single rod. ( e ) Fourier transform calculated from the monochrome real space image of ( c ) and ( d ). The colour bar indicates the logarithmic intensity scale. ( f ) Pair correlation function g( r ) found, from top to bottom, by calculating the g( r ) of a single frame, by calculating the g( r ) of the average of 150 frames, and from a perfect BCC lattice. The scale bars in ( a ) and ( c ) represent 10 μm, and in ( e ) represents 0.628 μm −1 . 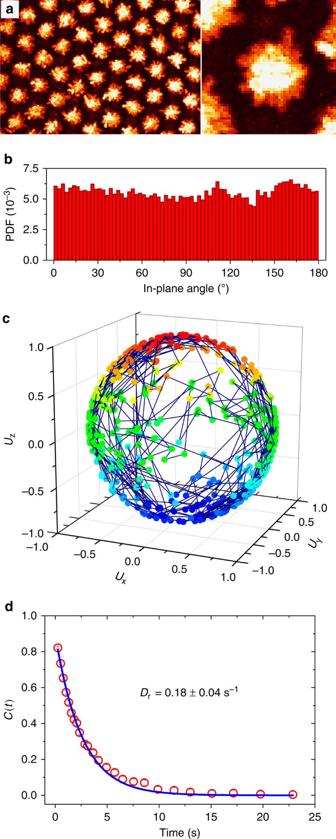Figure 2: Rotational dynamics. Silica rods R2 withϕ=0.005. (a) A superposition of 300 frames measured over 100.8 s and (b) the corresponding distribution of in-plane angles. (c) The rotational trajectory of a single rod on the unit sphere surface. (d) Orientational autocorrelation function versus timet. Full size image Figure 2: Rotational dynamics. Silica rods R2 with ϕ =0.005. ( a ) A superposition of 300 frames measured over 100.8 s and ( b ) the corresponding distribution of in-plane angles. ( c ) The rotational trajectory of a single rod on the unit sphere surface. ( d ) Orientational autocorrelation function versus time t . 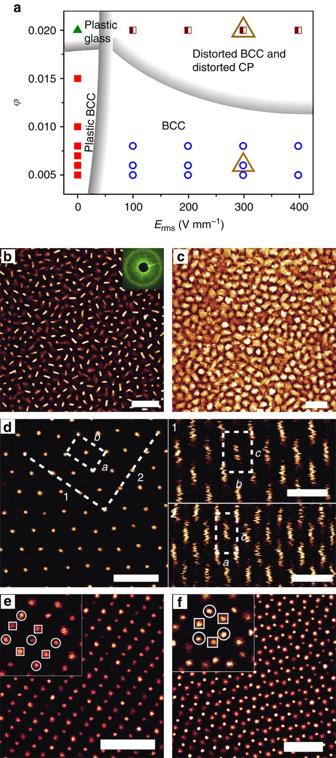Figure 3: Volume fraction-electric field phase diagram. Silica rods R2 withϕ=0.005~0.02. (a) The phase diagram. Thick grey lines indicate approximate phase boundaries. (b) Confocal image of a plastic glass phase; inset shows a 3D laser diffraction pattern. (c) A superposition of 120 frames of plastic glass measured over 98 s. (d) Confocal images of a fully BCC phase, left: (110) plane; top right: (001) plane; bottom right: (10) plane. The images for the (001) and (10) planes were reconstructed from the same x-y-z stack. (e) Distorted BCC phase and (f) distorted close packed phase atϕ=0.02, the focal plane is in between two neighbouring layers. In inset images, squares represent one layer, and circles represent one neighbouring layer. The scale bars from (b) to (f) represent 10 μm. Full size image Figure 3: Volume fraction-electric field phase diagram. Silica rods R2 with ϕ =0.005~0.02. ( a ) The phase diagram. Thick grey lines indicate approximate phase boundaries. ( b ) Confocal image of a plastic glass phase; inset shows a 3D laser diffraction pattern. ( c ) A superposition of 120 frames of plastic glass measured over 98 s. ( d ) Confocal images of a fully BCC phase, left: (110) plane; top right: (001) plane; bottom right: (10) plane. The images for the (001) and (10) planes were reconstructed from the same x-y-z stack. ( e ) Distorted BCC phase and ( f ) distorted close packed phase at ϕ =0.02, the focal plane is in between two neighbouring layers. In inset images, squares represent one layer, and circles represent one neighbouring layer. The scale bars from ( b ) to ( f ) represent 10 μm. 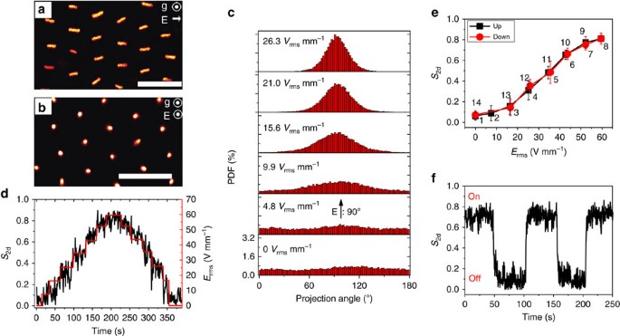Figure 4: Manipulation of the rotation using an external electric field. Silica rods R2 (a,b,d–f) and R3 (c) withϕ=0.005. (a,b) Confocal images of the rods oriented by different field directions. (c) In-plane angular distribution of rods on a crystal lattice as a function of field strength. (d) Nematic order parameter (2D) and corresponding field strength as a function of time. (e) Nematic order parameter (2D) versus field strength, showing the absence of hysteresis. The designated time points were 0, 14, 35, 65, 89, 133, 161, 188, 228, 253, 286, 310, 340, 355 s. The vertical error bars are the s.d. of the calculated values displayed. (f) Fast switching between the on-state (same orientation) and off-state (random orientation). The scale bars in (a) and (b) represent 10 μm. Full size image Figure 4: Manipulation of the rotation using an external electric field. Silica rods R2 ( a , b , d – f ) and R3 ( c ) with ϕ =0.005. ( a , b ) Confocal images of the rods oriented by different field directions. ( c ) In-plane angular distribution of rods on a crystal lattice as a function of field strength. ( d ) Nematic order parameter (2D) and corresponding field strength as a function of time. ( e ) Nematic order parameter (2D) versus field strength, showing the absence of hysteresis. The designated time points were 0, 14, 35, 65, 89, 133, 161, 188, 228, 253, 286, 310, 340, 355 s. The vertical error bars are the s.d. of the calculated values displayed. ( f ) Fast switching between the on-state (same orientation) and off-state (random orientation). The scale bars in ( a ) and ( b ) represent 10 μm. 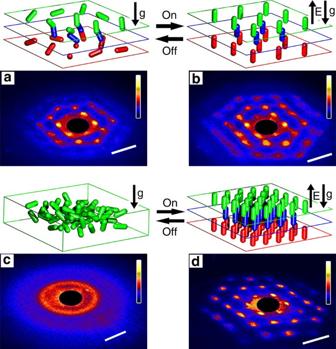Figure 5: Laser diffraction patterns of crystal switching. The field was perpendicular to the projection plane. Silica rods: R2. (a) Plastic crystal and (b) fully crystalline state of the silica rods atϕ=0.006, see the highlight with a triangle inFig. 3a; (c) plastic glass and (d) a fully crystalline state of the silica rods atϕ=0.02, see the highlight with a triangle inFig. 3a. The scale bar is 2 cm. The projection plane wasca. 11 cm behind the sample. The color bar indicates the scattering intensity scale. Full size image Figure 5: Laser diffraction patterns of crystal switching. The field was perpendicular to the projection plane. Silica rods: R2. ( a ) Plastic crystal and ( b ) fully crystalline state of the silica rods at ϕ =0.006, see the highlight with a triangle in Fig. 3a ; ( c ) plastic glass and ( d ) a fully crystalline state of the silica rods at ϕ =0.02, see the highlight with a triangle in Fig. 3a . The scale bar is 2 cm. The projection plane was ca . 11 cm behind the sample. The color bar indicates the scattering intensity scale. Full size image Plastic crystal structure As Fig. 1 shows in detail, the 3D lattice on which the rods rotate is indeed of BCC symmetry ( Fig. 1a–f and Supplementary Figs 1 and 2 ). In addition, it is clear that the softness of the inter-particle potential as well as the rotations of the individual rods on their 3D lattice makes visual identification of the actual structure from (sets of) individual images relatively hard. However, as a testament to the true 3D long-ranged periodicity and stability of these crystals, an average of 150 frames taken over 5 min produced an almost perfect lattice: half of this time series is shown as a frame-averaged image in Fig. 1c , and the other half as in-plane trajectories in Fig. 1d ( Supplementary Movies 1, 2 ). The combination of Fig. 1c and d demonstrates the restricted Brownian translational motion of the rods to lattice sites in the plastic BCC phase. The sharp peaks from first to even fifth order in the corresponding Fourier transform shown in Fig. 1e illustrate the nearly perfect crystallinity present even over the relatively long averaging period. We further illustrated the softness and the positional order of the crystal with two-dimensional (2D) pair correlation functions g( r ) ( Fig. 1f ) with (red) and without averaging (blue). The peaks from the time-averaged image match well with a perfect (110) plane of a BCC phase (black). The position of the first peak at 2.2 times the length of the rods again illustrates the long range repulsion between the rods. The resulting extremely low effective mass density of these crystals explains why gravity hardly affected the lattice spacing as a function of height in the samples studied. Unfortunately, a theoretical description of systems of anisotropic particles with electrostatic double layers the size of the particles is not available yet as the inter-particle interactions are quite difficult to solve [21] . Rotational dynamics We explored the nature of the rotational motion of the rods on their BCC lattice and investigated whether rods influence each other’s rotation at the lowest volume fractions ϕ ~0.005. In Fig. 2a , we show the superposition of a time sequence of 300 frames taken over 100.8 s. Already from the symmetry of the pattern, we can reasonably infer that the rods explore all the orientations. This is confirmed by the absence of structure in the orientation distribution of the rods as projected in the 2D imaging plane ( Fig. 2b ). To further verify the free rotation of the rods, we also measured a 3D rotational trajectory of a single rod on its lattice position by extracting its angular coordinates from a time series of images in x-y-z-t scanning mode ( Fig. 2c , Methods). The orientation distribution on the unit sphere is homogeneous, showing that the rod explores all orientations ( Supplementary Movie 2 ). From an average of all the trajectories of 35 rods, we obtained the rotational autocorrelation function C ( t ) and, by fitting this function ( Fig. 2d , Methods), the rotational diffusion coefficient: D r =0.18±0.04 s −1 . This value is close to the theoretical value for a free rod 0.19 s −1 . When ϕ was increased above 0.005 the plastic crystalline behaviour was still observed, although the (almost) free rotations demonstrated in Fig. 2 became more and more influenced by neighbouring particles. Interestingly though, not the rotational degrees of freedom were lost when ϕ was increased above roughly 0.018, but it was the positional order that was lost ( Fig. 3a ). This loss of positional order, without translational diffusion, but with significant rotational mobility is clearly seen by comparing Fig. 3b and c with Fig. 1c and d . As will be shown below ( Fig. 5 ), this transition to a ‘plastic glass’ was also apparent in scattering experiments where liquid like order was demonstrated similarly as shown in the inset of Fig. 3b . In Supplementary Movie 3 the rotations of many of the rods can be clearly observed, while positionally there is no relaxation. This plastic glass phase is a remarkable demonstration of the decoupling of the glass transitions of the positional and rotational degrees of freedom, as has been discussed earlier based on simulations and theory (for examples, see refs 22 , 23 , 24 ). The ability to follow the 3D rotations of the particles quantitatively in real space gives unprecedented possibilities to study this new type of glass transition, work on which is on-going. Moreover, the positional glass can be reversibly switched to a crystalline state by an external electric field as will be demonstrated below. Alignment under an electric field Electric fields are known to couple strongly to the alignment of liquid crystal phases enabling many applications [9] . To examine whether the particle orientations in plastic crystals can also be controlled, we applied a homogeneous external electric field with a frequency of 1 MHz so that the double layer is not able to follow the field and only effects of dielectric polarization of the particles remain [6] . Because the long range of the particle repulsion, coupling of induced dipoles between particles is significantly weaker than the thermal energy at almost all field strengths used, so in the systems studied here induced dipoles couple only to the external field ( Supplementary Note 1 , Supplementary Figs 3–5 and Supplementary Tables 1–3 ). Nevertheless, as shown qualitatively in Fig. 3 and quantitatively in Fig. 4 , fields of sufficient strength align the rods, fully arresting the rotational freedom of the plastic crystals, thus switching from a plastic crystal to a fully ordered 3D crystalline state ( Fig. 4a,b ). As expected from the lack of dipole-dipole coupling ( Supplementary Note 1 ), the lattice symmetry and spacing are preserved in this transition as illustrated in Fig. 3d and Supplementary Movie 4 . To investigate the nature of the transition from a plastic to a full BCC crystal, we quantified the projected angular distributions measured by taking 2D time series of (110) crystal planes ( Fig. 4c , ϕ =0.005) as a function of the electric field strength with the field parallel to the imaging plane ( Fig. 4a ). Already at a field strength of 25 V rms mm −1 , the rotations became highly restricted ( Fig. 4c ). However, there was no indication of a sudden jump in the angular distribution or the nematic order parameter S 2d of in-plane angles, indicating that the transition as a function of the field was continuous at this volume fraction (Methods). This is also borne out by the absence of any hysteresis when the field was slowly cycled from low to high values and back ( Fig. 4d,e ). At a higher volume fraction ( ϕ =0.02), where rotational coupling between neighbouring rods becomes more apparent, we observed a slight hysteresis in the switching curve. Figure 4f gives an indication of the switching speed. When the field is switched on/off instantaneously, it takes a few seconds to achieve full alignment of the rods ( Supplementary Movie 5 ). Fully in line with expectations, such switching did not affect the crystallinity. At higher volume fractions ( ϕ φ0.015) and for field strengths where the positional order was not lost, we observed a relatively large region where distorted BCC crystal ( Fig. 3a,e and Supplementary Fig. 6 ) was found mixed with crystals with a different stacking and symmetry (compare Fig. 3e,f ). These other crystals were similar to those observed for hard spheres: randomly stacked close packed (CP) layers ( Supplementary Fig. 6 ). There was not a sharp transition region in the phase diagram between BCC and the randomly close packed layers, quite similar to the case reported for spheres in a similar inter-particle distance range [25] . As mentioned, there are unfortunately no simulations or theory for comparison. It is also quite intriguing that at the higher volume fractions and relatively low field strengths there is a transition between the already mentioned plastic glass and a 3D fully crystalline state that is completely reversible. Apparently and intriguingly, without a field the plastic glass is more stable than the crystal. Light diffraction Because of possible applications of plastic crystals in photonics, we also investigated the switching of both the plastic glass phase and the plastic BCC crystals into their fully crystalline counterparts by light scattering. Figure 5a,b demonstrates the change in scattering pattern when switching between a plastic and fully crystalline BCC state. The only change between these two states is the presence or absence of (almost) free rotations as depicted in the schematics above the scattering patterns. Consequently, the Bragg peaks stayed at the same location, although there was a significant increase in intensity of the peaks moving from the plastic to the crystalline state. In the Supplementary Note 2 we show how the form factor of the rods explains this difference. Although the silica rods had a refractive index close to that of the solvent, their large size meant that their scattering was a strong function of their orientation with respect to the incident light ( Supplementary Note 2 and Supplementary Fig. 7 ). The resulting difference in form factor explains the increase in the higher order Bragg peaks ( Supplementary Fig. 8 ). As mentioned, the time scale of the change in the scattering pattern was on the order of a few seconds ( Fig. 4 ). Switching between the plastic glass ( Fig. 5c ) and the distorted BCC crystal ( Fig. 5d ) is clearly more marked because the structure factor switches between that of a liquid and that of a crystal. However, the increase in switching time is also marked: it took approximately 10 min to switch between these two states. However, the interest in this case lies perhaps not in a photonic application, but more in the fact that it is quite intriguing to be able to reversibly switch between a (positionally) glassy state and a fully 3D crystalline state with an external field. Presently, work is in progress to fully characterize this transition on the single-particle level. More quantitative information on the rotations can be obtained for slower rods by increasing the solvent viscosity [26] . Because the rods studied here are quite long and their aspect ratio is quite high, we expect that switchable plastic crystals can be obtained with a broad range of other monodisperse anisotropic particles in combination with sufficiently long-ranged charged repulsions. Such repulsions can be achieved in a large range of solvents but should be accessible also in water for anisotropic particles of a smaller size. It is quite clear that the systems studied here were not yet optimized for applications. For instance, clear improvements in switching speed by going to smaller rods and a much more marked photonic switching will be possible, for instance, with gold rods, which are known to have two strongly different plasmonic resonances excitable by changing the orientation of the rods [27] . As another example, rod-like superparticles built up from nanorods with strongly anisotropic luminescent light emission have recently been realized as well [28] . Results on other rod-like systems have already indicated that at lower electric field frequencies a phase diagram as studied here will become richer as a result of strong coupling of the double layers to the external field [29] . Finally, the demonstrated ability to quantitatively analyse rotations on the single particle level in strongly interacting systems will no doubt lead to new insights into the role played by rotations in fundamental processes such as crystallization and the glass transition. Particle synthesis The fluorescent silica rod-like particles were prepared by a two-step procedure. In the first step, we prepared monodisperse silica rods following a reported procedure [18] . Thirty grams of poly(vinylpyrrolidone) (PVP, M n =40.000, Sigma-Aldrich) was dissolved in 300 ml of 1-pentanol (99%, Sigma-Aldrich) containing 30 ml of absolute ethanol (Baker). After PVP was dissolved, 8.4 ml of ultrapure water (18.2 MΩ), 2 ml of 0.18 M sodium citrate dihydrate (99%, Sigma-Aldrich) and 6.75 ml of ammonia aqueous solution (25%, Merck) were added and the flask was shaken. Afterwards, 2.5–4.5 ml of tetraethylorthosilicate (TEOS, 98%, Sigma-Aldrich) was added. The mixture was shaken and then allowed to react undisturbed for 24 h. The as-prepared silica rods were separated by centrifuge and then washed with ethanol, water and ethanol, respectively. To grow a fluorescent shell, half of the as-prepared silica rods were dispersed into 150 ml ethanol containing 10 ml of water and 12 ml of ammonia aqueous solution (25%). Then 5 ml of a solution containing 0.8 ml TEOS, 25 mg of fluorescein isothiocyanate (FITC, isomer I, 90%, Sigma-Aldrich) and 37 μl of 3-aminopropyltriethoxysilane (APS, 99%, Sigma-Aldrich) was added. The reaction was stirred overnight. Afterwards, the silica rods were washed with ethanol three times. To grow a non-fluorescent shell, a similar procedure was performed but without the addition of FITC and APS. The thickness of the shell was adjusted by controlling the amount of added TEOS (0.5–2 ml). The as-prepared colloidal rods have a three-layered structure: non-fluorescent silica core, fluorescent shell (dye: FITC, ca . 30–50 nm) and non-fluorescent shell ( ca . 100 nm). In the second step, we modified the silica rods with octadecyltrimethoxylsilane (OTMOS, 90%, Sigma-Aldrich) by ultrasonic-assisted coating procedure. In brief, a solution of OTMOS, butylamine (BA, 99.5%, Sigma-Aldrich) and dried toluene (1:1:10 v/v/v) was prepared, and then 10 (wt) % of dried silica rods was added to this solution. The suspension was sonicated at 30~55 °C for 4 h (Branson 2250). Afterwards, the colloidal rods were washed in turn with toluene, cyclohexane and cyclohexylchloride (CHC, >98%, Merck). Finally, the colloidal rods were dispersed in deionized CHC for further use. We used three sizes of fluorescent colloidal silica rods, named R1, R2 and R3. R1: L =2.36 μm (6.3%), D =0.58 μm (10.6%), L / D =4.1; R2: L =2.29 μm (6.0% ), D =0.60 μm (6.5%), L / D =3.8; R3: L =3.30 μm (6.3%), D =0.59 μm (8.7%), L / D =5.6. Here L and D are the mean length and diameter with the polydispersity (standard deviation divided by the mean) between parentheses. Sample preparation The sample suspension medium was CHC. The received CHC (conductivity>>1,000 pS cm −1 ) was deionized by using molecular sieves (4 Å, Aldrich) and subsequent neutral aluminium oxide (Aldrich). After purification, CHC had a conductivity as low as around 5–10 pS cm −1 . Rectangular capillaries (0.1 × 1 mm 2 , 0.1 × 2 mm 2 , 0.5 × 0.5 mm 2 , VitroCom, UK) were used as the sample cells. Electrodes consisting of a 3 nm layer of Cr and a 6–10 nm layer of Au were sputter-coated on two opposing outer surfaces of these capillaries and connected to a function generator and amplifier. The sample capillary was then fixed on a glass slide and sealed with UV-cured glue (Norland, No. 68). Confocal microscopy measurement The samples were studied with a laser scanning confocal microscope (Leica TCS SP2 and Leica TCS SP8 equipped with a 12,000 kHz resonant scanner). All images were taken in fluorescence mode. The excitation wavelength was 488 nm. To obtain 3D data sets, care was taken to ensure that rods did not move or rotate too much during the collection of an x-y-z-t set. The measured rotational diffusion time was 2.78 s for sample R2. The scanning time of each series was 0.26 s, achieved by scanning 304 × 100 × 18 pixels with a pixel size of 178 nm in x-y and 396 nm in z, for which we achieved angular coordinates with an uncertainty estimated to be around 24°. The extraction of the positional and the angular coordinates of the rod-like particles was done using a homemade computer tracking code. Rod-like particle tracking We identified both the positions and the orientations of rod-like particles in 2D confocal microscopy images or 3D confocal image data sets. To achieve this, two feature-finding algorithms were written that identify the backbone (main axis) of rod-like particles in two and three dimensions. In brief, both algorithms consisted of five steps. (1) Filtering out noise in the confocal microscopy images. A Gaussian blur was applied and a certain amount of (background) intensity was subtracted from the images. (2) Identifying the candidate backbone pixels of the rods. We checked if pixels brighter than a certain threshold value formed a line in the image. (3) Backbone pixels were connected and ordered into clusters. (4) For every cluster a line segment was fitted to the pixels in the neighbourhood of this cluster. From this line, the position and orientation of the particle were extracted. (5) Filtering out misidentified or out of focus particles based on length and intensity. Supplementary Fig. 9 shows an example of the 2D identification of rod-like particles in a BCC phase. The white lines show the identified main axis of the rods, from which the projected 2D positions and orientations of the particles were obtained. The trajectories of the centre of mass and the orientations of rods were obtained by an Interactive Data Language (IDL) routine based on the particle tracking programs of Crocker and Grier [30] . To uniquely track the tip of the (nearly up-down symmetric) rod, it is required that the rotation angle of individual rods between successive frames was less than π /2. It was verified that the rotations larger than π /2 were negligible at a time-step of 0.26 s. Electrical conductivity measurement We estimated the Debye screening length by measuring the conductivity of the deionized solvent CHC with a Scientifica 627 conductivity meter. For the calculation of ionic strength, we made use of Walden’s rule [6] , [31] , which states that the product of the limiting equivalent conductance and the viscosity is a constant between different media, that is, Λ 0 Ethanol η 0 Ethanol = Λ 0 CHC η 0 CHC . We used literature values for the limiting equivalent conductance of HCl in ethanol [32] and the viscosity of 1.5675, mPa.s for CHC [33] . The Debye screening length can then be estimated by Here, λ B =e 2 /(4 πεε 0 k B T ) is the Bjerrum length, and ε and ε 0 are the dielectric constant of the solvent and the permittivity of vacuum. e is the elementary charge, k B is Boltzmann’s constant and T is the absolute temperature. A final conductivity of ca . 10 pS cm −1 for particle-free CHC corresponded to κ −1 of ca . 5 μm estimated by the above formula. Electrophoretic mobility measurements To estimate the surface charge of our particles, we measured the electrophoretic mobility of a diluted suspension sample ( ϕ =0.0005) by confocal microscopy [34] . The sample cell was a 0.1 × 2 mm 2 capillary cell with two parallel 50-μm-diameter nickel-alloy wires running along the side walls. We filled the cell with our sample and sealed it with UV-glue. The stationary layer z axis position was calculated as described before [34] . In a direct current field, the motion of particles in the stationary layer was recorded as a time series of images. From the mobility we then obtained the zeta potential using the Hückel equation, which applies to ideal diluted suspensions with large Debye screening length. Laser light diffraction A 543.5 nm green HeNe laser was shone through the horizontal capillary cell. Diffracted light was collected on a white paper screen placed about 11–16 cm behind the sample. Pictures were taken with a digital camera at an angle of around 50 degrees to the normal. Rotational auto-correlation function The rotational auto-correlation function is defined as: where N is the number of the particles in the system, u i is the unit vector that defines the orientation of particle i , and the angular brackets denote the canonical average. The angular coordinates of the rods are obtained from 3D tracking of confocal image data sets (x-y-z-t). The rotational auto-correlation function was calculated by averaging over 35 particles over 494 time steps. The auto-correlation function was then fitted to the expression to obtain the rotational diffusion coefficient D r =0.18±0.04 s −1 for silica rods R2 at ϕ =0.005. The expression is derived from the equation for the mean squared angular displacement used in ref. 35 . Here, ε r 2 is a term accounting for the statistic error in measurements of u i (t) and τ is the exposure time (the scanning time of a x-y-z data set). The error ∈ r is estimated to be 0.42 by the fitting, which corresponds to an uncertainty in the identification of u i ( t ) of 24°. For comparison, a theoretical rotational diffusion coefficient for a freely rotating cylinder in a dilute suspension was calculated via [36] where L is the length of the rod, D the diameter, k B the Boltzmann constant, T =294 K the temperature and η 0 =1.57 mPa the viscosity of the solvent. δ ⊥ is for the correction of end effects. The calculated D r of rods R2 is 0.19 s −1 which is within the range of our experimental measurement for rods with long-ranged repulsion rotating in a plastic crystal. Orientational order parameter. The 2D nematic order parameter S 2d is defined as: where N is the number of particles in the image, θ is the angle with respect to the nematic director and the angular brackets denote the canonical average. We determined the order parameter and director by finding the eigenvalues and eigenvectors of the second rank tensor Q. where u i is unit vector in the direction of the long axis of the i th rod, δ αβ is Kronecker delta. The order parameter is the positive eigenvalue of Q αβ , and the director is the eigenvector associated with the corresponding eigenvalue. How to cite this article: Liu, B. et al. Switching Plastic Crystals of Colloidal Rods with Electric Fields. Nat. Commun. 5:3092 doi: 10.1038/ncomms4092 (2014).